The first total synthesis of the cyclodepsipeptide pipecolidepsin A Pipecolidepsin A is a head-to-side-chain cyclodepsipeptide isolated from the marine sponge Homophymia lamellosa . This compound shows relevant cytotoxic activity in three human tumour cell lines and has unique structural features, with an abundance of non-proteinogenic residues, including several intriguing amino acids. Although the moieties present in the structure show high synthetic difficulty, the cornerstone is constituted by the unprecedented and highly hindered γ-branched β-hydroxy-α-amino acid D -allo -(2 R ,3 R ,4 R )-2-amino-3-hydroxy-4,5-dimethylhexanoic acid (AHDMHA) residue, placed at the branching ester position and surrounded by the four demanding residues L -(2 S ,3 S ,4 R )-3,4-dimethylglutamine, (2 R ,3 R ,4 S )-4,7-diamino-2,3-dihydroxy-7-oxoheptanoic acid, D -allo -Thr and L -pipecolic acid. Here we describe the first total synthesis of a D -allo -AHDMHA-containing peptide, pipecolidepsin A, thus allowing chemical structure validation of the natural product and providing a robust synthetic strategy to access other members of the relevant head-to-side-chain family in a straightforward manner. Marine sponges are a relevant source of biologically active compounds. Among these, depsipeptides and cyclodepsipeptides stand out for their broad spectrum of biological activities and structural diversity [1] , [2] , [3] . The presence of several unique residues and the complex structural features shown by these natural products make their structural elucidation challenging. However, given the interesting therapeutic profiles of these compounds, research in this field has thrived over recent years, and several depsipeptides are now undergoing evaluation in clinical trials. In 2010, one of our groups described three new cyclodepsipeptides, named pipecolidepsin A–C [4] , isolated from the marine sponge Homophymia lamellosa collected on the coasts of Madagascar. Pipecolidepsins belong to a growing class of peptides that have a unique structural template, namely a head-to-side-chain arrangement via an ester bond, in which the N -terminus has been blocked with a polyketide moiety. A head-to-side-chain peptide is a cyclic peptide in which the macrocyclization happens to occur between the C -terminus and a side chain. This β-branched framework, which characterizes all the members of this new class of non-ribosomal cyclodepsipeptides [5] , comprises the following: a 22- or a 25-membered macrolactone; the presence of complex and rare amino acids; a branching position occupied by a D -allo -β-hydroxy-α-amino acid acylated by the unique (2 S ,3 S ,4 R )-3,4-dimethylglutamine (diMeGln) residue; and an N -terminus coupled to a saturated or unsaturated β-hydroxy acid. Examples of members of this family include callipeltin A [6] , papuamides [7] , [8] , neamphamides [9] , [10] , [11] , theopapuamides [12] , [13] , mirabamides [14] , [15] and homophymines [16] , [17] . Of note, all of them show relevant therapeutic profiles, mostly including potent cytotoxic and anti-HIV activities. The same topology of head-to-side-chain cyclodepsipeptide is also present in other peptides isolated from cyanobacteria and mollusks. However, the uniqueness of the residues present in the peptides isolated from marine sponges and, therefore, the complexity of their total synthesis represent a differential trait. The residue placed at the branching position of the head-to-side-chain cyclodepsipeptides has a key structural role as its β-hydroxyl group allows the β-branched arrangement. D -allo -Thr is the most frequent amino acid; nevertheless, pipecolidepsin A and B and homophymines bear the unprecedented and extremely hindered D -allo -(2 R ,3 R ,4 R )-2-amino-3-hydroxy-4,5-dimethylhexanoic acid (AHDMHA) at the same position. This amino acid represents the cornerstone for the synthesis of pipecolidepsin A, as it is involved in the ester bond and is surrounded by demanding moieties. Thus, D -allo -AHDMHA acylates the β-branched D -allo -Thr; its N α is acylated by the diMeGln; and its β-hydroxy function is esterified by the N -alkyl-α-amino acid L -pipecolic acid. Furthermore, the amino function of the diMeGln moiety is acylated by the bulky γ-amino-α,β-dihydroxy acid, (2 R ,3 R ,4 S )-4,7-diamino-2,3-dihydroxy-7-oxoheptanoic acid (DADHOHA). These five residues comprise the synthetic core of pipecolidepsin A ( Fig. 1 ). Finally, the macrocyclic region also contains rare and bulky amino acids, such as L -threo -β-EtO-Asn and L - N Me-Gln, and the exocyclic arm is terminated by the β-hydroxy acid (2 R ,3 R ,4 R )-3-hydroxy-2,4,6-trimethylheptanoic acid (HTMHA). 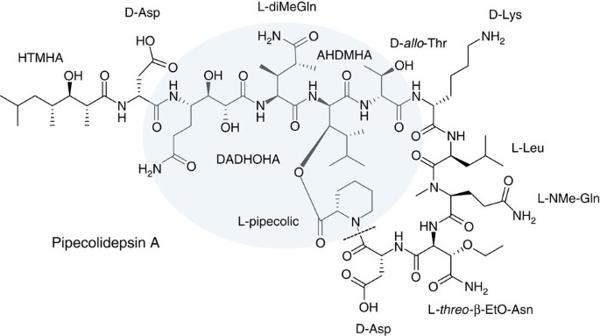Figure 1: Chemical structure of pipecolidepsin A. The synthetic core is highlighted in blue and the cyclization point with a dashed line. Figure 1: Chemical structure of pipecolidepsin A. The synthetic core is highlighted in blue and the cyclization point with a dashed line. Full size image The synthesis of this kind of peptide is hampered by the presence of several exotic non-commercial residues and the construction of the synthetic core centred at the D -allo -AHDMHA building block. The consecutive assembly of the rare amino acids, usually N -alkyl and β-branched residues, is translated into poor acylation rates and unexpected side reactions, and the building of the ester linkage is always a synthetic challenge, especially in an exceptionally hindered environment such as that of pipecolidepsin A. Despite the major synthetic challenges, the difficult access to natural sources of this kind of product, their pharmacological significance and the necessity for chemical structure validation have encouraged the development of robust synthetic strategies that overcome the high complexity mentioned previously, supplying large enough amounts of the product to perform more detailed biological studies. Here we describe the first total synthesis of a head-to-side-chain cyclodepsipeptide bearing the D -allo -AHDMHA residue at the branching position. A full solid-phase approach was established, allowing rapid access to analogs, thus providing further insight into the crucial structure-activity relationships required for these molecules to proceed in a medicinal chemistry program. Synthesis of Fmoc-DADHOHA(acetonide,Trt)-OH Before the peptide assembly on solid phase, several of the component residues of target 1 were synthesized. New routes were developed for Fmoc- L -threo -β-EtO-Asn(Trt)-OH [18] , Fmoc-DADHOHA(acetonide,Trt)-OH and Fmoc- D -allo -AHDMHA-OH, whereas synthetic strategies to access Fmoc- N Me-Gln-OH [19] , Fmoc-diMeGln-OH [20] , [21] , and HTMHA [22] ( Supplementary Fig. S1 ) were adapted from published protocols. Excluding Fmoc- L -threo -β-EtO-Asn(Trt)-OH and Fmoc-DADHOHA(acetonide,Trt)-OH, the rest of the building blocks were prepared with unprotected side chains. Z- L -Gln(Trt)-OH was converted into the Weinreb amide using 1-ethyl-3-(3-dimethylaminopropyl)carbodiimide (EDC) and 1-hydroxybenzotriazole (HOBt) and then reduced to the corresponding aldehyde using AlLiH 4 with a 93% yield over the two steps. At this point, a cis -stereospecific Horner–Wadsworth–Emmons olefination, using a Still–Gennari phosphonate in the presence of KHMDS, allowed the transformation of the initial α-amino acid into a γ-amino acid (67% yield). Cis -disubstituted olefins are poor substrates for asymmetric dihydroxylation [23] , cis -allylic and homo-allylic alcohols being the exception. Some improvements have been reported with cyclic cis -disubstituted olefins; however, the enantiomeric excess described for acyclic and non-conjugated olefins are not satisfactory [24] , [25] . Thus, alkene 5 was subjected to dihydroxylation with catalytic OsO 4 and a stoichiometric amount of NMO as the oxidant to provide, after purification, the two diastereomeric diols with 38% and 39% yield. The diols were protected as pentacyclic acetals in the presence of acetone dimethyl acetal and catalytic PPTS, and then subjected to basic hydrolysis of the methyl ester and hydrogenolysis of the Z group. The last Fmoc-protection step proceeded with moderate yields (46% and 45% yield for the two diastereomers) as a result of a spontaneous intramolecular lactamization side reaction that occurred in all the conditions tested. Final building block 10 for solid-phase peptide synthesis was obtained in 15% overall yield after eight steps ( Fig. 2 ). To accomplish the total stereochemical determination of the building block, the synthesis of a more rigid structure that would allow its assignation based on nuclear overhauser effect (NOE) cross-peaks analysis was required [26] . Hence, the bicyclic structure 11 was synthesized by reacting intermediate 9 with EDC and HOBt. Interpretation of NOE cross-peaks led to univocal assignment of the absolute configuration for C2 and C3 ( Supplementary Fig. S2 ). 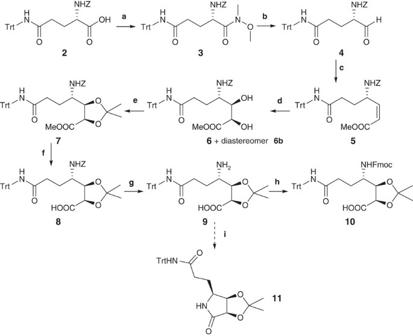Figure 2: Synthesis of Fmoc-DADHOHA(acetonide,Trt)-OH. (a) EDC, HOBt and dry DMF, 25 °C, 30 min;N,O-dimethylhydroxylamine, DIEA and dry DMF, 25 °C, 3 h, 96%; (b) LiAlH4and dry THF, 0 °C, 30 min, 97%; (c) (CF3CH2O)2P(O)CH2CO2Me, KHMDS, 18-crown-6 and dry THF, −78 °C, 3 h, 67%; (d) catalytic OsO4, NMO and THF−H2O (9:1), 25 °C, 10 days, 38% (6) and 39% (diastereomer6b); (e) (CH3)2C(OCH3)2, catalytic PPTS, dry toluene, 25→50 °C, 36 h, 77% (7) and 96% (diastereomer7b); (f) LiOH, THF−H2O (9:1), 0 °C, 2 h, 98% (8) and 96% (diastereomer8b); (g) H2(1 atm), Pd-C (10%), dry MeOH, 25 °C, 5 h, 94% (9) and 93% (diastereomer9b); (h) Fmoc-Cl, NaN3, dioxane−H2O (1:1), pH 9, 0 °C, 5 days, 46% (10) and 45% (diastereomer10b); and (i) EDC, HOBt and DMF, 25 °C, 6 h, 52% (11) and 61% (diastereomer11b). Figure 2: Synthesis of Fmoc-DADHOHA(acetonide,Trt)-OH. ( a ) EDC, HOBt and dry DMF, 25 °C, 30 min; N,O -dimethylhydroxylamine, DIEA and dry DMF, 25 °C, 3 h, 96%; ( b ) LiAlH 4 and dry THF, 0 °C, 30 min, 97%; ( c ) (CF 3 CH 2 O) 2 P(O)CH 2 CO 2 Me, KHMDS, 18-crown-6 and dry THF, −78 °C, 3 h, 67%; ( d ) catalytic OsO 4 , NMO and THF−H 2 O (9:1), 25 °C, 10 days, 38% ( 6 ) and 39% (diastereomer 6b ); ( e ) (CH 3 ) 2 C(OCH 3 ) 2 , catalytic PPTS, dry toluene, 25→50 °C, 36 h, 77% ( 7 ) and 96% (diastereomer 7b ); ( f ) LiOH, THF−H 2 O (9:1), 0 °C, 2 h, 98% ( 8 ) and 96% (diastereomer 8b ); ( g ) H 2 (1 atm), Pd-C (10%), dry MeOH, 25 °C, 5 h, 94% ( 9 ) and 93% (diastereomer 9b ); ( h ) Fmoc-Cl, NaN 3 , dioxane−H 2 O (1:1), pH 9, 0 °C, 5 days, 46% ( 10 ) and 45% (diastereomer 10b ); and ( i ) EDC, HOBt and DMF, 25 °C, 6 h, 52% ( 11 ) and 61% (diastereomer 11b ). Full size image Synthesis of Fmoc-AHDMHA-OH The γ-branched carbon skeleton of the unique AHDMHA moiety was set up by reaction of Garner’s aldehyde 12 with 2-lithio-3-methyl-2-butene in moderate yields (36%). Hydrogenation of the tetra-substituted olefin 13 in the presence of catalytic Pd-C proceeded smoothly and with excellent stereoselectivity when performed on this diastereomer. All attempts to cleave the acetonide-protecting group were inappropriate. Finally, an intramolecular triflate-mediated cyclization with inversion [27] , involving the Boc-group and the hydroxyl function, provided a bicyclic structure that allowed selective cleavage of the acetonide group by means of a Jones oxidation. The resulting cyclic carbamate 16 , obtained with a 60% yield after two steps, was then hydrolysed by refluxing aqueous HCl to quantitatively give the free amino acid as a hydrochloride, which underwent a final Fmoc protection to furnish the appropriate building block 18 for solid-phase peptide synthesis in 15% overall yield after six steps ( Fig. 3 ) [28] . Absolute configuration of all the stereocenters of diastereomer 17 was confirmed by X-ray ( Supplementary Fig. S3 and Supplementary Tables S1–S5 ). 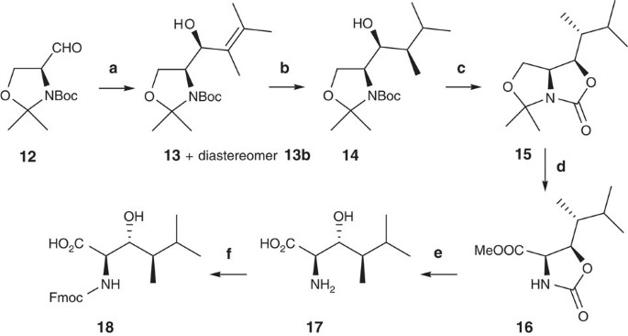Figure 3: Synthesis of (2R,3R,4R)-Fmoc-D-allo-AHDMHA-OH. (a) i. 2-bromo-3-methyl-2-butene,tBuLi, Et2O, −78 °C, 3.3 h; ii. Garner’s aldehyde12, Et2O, −78→25 °C, 1.2 h, 36%; (b) H2(4 atm), Pd-C (10%), MeOH, 25 °C, 2 days, 78%; (c) 2,6-di-tert-butyl pyridine, Tf2O, DCM, 0 °C, 10 min, 90%; (d) i. Jones reagent, acetone, 0 °C, 15 h; ii. Diazomethane, Et2O, 67%; (e) Concentrated HCl, reflux, 72 h, 100%; and (f) Fmoc-OSu, Na2CO3, H2O−dioxane (1:1), 25 °C, 15 h, 91%. Figure 3: Synthesis of (2 R ,3 R ,4 R )-Fmoc- D - allo -AHDMHA-OH. ( a ) i. 2-bromo-3-methyl-2-butene, t BuLi, Et 2 O, −78 °C, 3.3 h; ii. Garner’s aldehyde 12 , Et 2 O, −78→25 °C, 1.2 h, 36%; ( b ) H 2 (4 atm), Pd-C (10%), MeOH, 25 °C, 2 days, 78%; ( c ) 2,6-di-tert-butyl pyridine, Tf 2 O, DCM, 0 °C, 10 min, 90%; ( d ) i. Jones reagent, acetone, 0 °C, 15 h; ii. Diazomethane, Et 2 O, 67%; ( e ) Concentrated HCl, reflux, 72 h, 100%; and ( f ) Fmoc-OSu, Na 2 CO 3 , H 2 O−dioxane (1:1), 25 °C, 15 h, 91%. Full size image Solid-phase synthesis of pipecolidepsin A With all the building blocks in hand, we undertook the solid-phase synthesis of pipecolidepsin A ( Fig. 4 ). First of all, low-functionalized aminomethyl resin (0.36 mmol g −1 of resin) was properly derivatized with the 3-(4-hydroxymethylphenoxy)propionic acid (AB linker) using HBTU/HOBt/DIEA in dimethylformamide (DMF) for 1.5 h. Then, the linear precursor assembly started by side-chain anchoring of Fmoc- D- Asp(OH)-OAllyl employing DIPCDI and DMAP in DMF−DCM for 3 h. The treatment was repeated twice. The Allyl protection of the α-carboxyl function was chosen for being orthogonal to the Fmoc and t Bu groups, thereby allowing macrolactamization on solid phase. The peptide elongation proceeded smoothly using HATU/HOAt/DIEA in DMF for 1 h until incorporation of the (2 R ,3 R ,4 R )-Fmoc- D -allo -AHDMHA-OH residue, furnishing the heptapeptide with 91% purity, where the main impurity was the dehydrated by-product at the N Me-Gln residue ( Fig. 4 ). Only Fmoc-Leu-OH required re-coupling. At this point, Fmoc-diMe Gln-OH was introduced using DIPCDI/HOBt (without pre-activation) in DMF for 1 h to minimize the dehydration side reaction down to a reasonable 11%. Keeping this Fmoc in its place, the ester bond was constructed under fine-tuned conditions using Alloc–pipecolic–OH (15 eq. ), DIPCDI (15 eq. ), DMAP (0.5 eq. ), DCM–DMF (9:1), 45 °C, for 2.3 h, providing quantitative conversions and keeping the epimerization to an acceptable 11%, taking into account the highly hindered system. The side product was successfully removed in the final purification. A short Fmoc-deprotection (2 × 2 min) was followed by an efficient and rapid incorporation of the (2 R ,3 R ,4 S )-Fmoc-DADHOHA(acetonide,Trt)-OH moiety by means of HATU/HOAt/DIEA in DMF with 1 min of pre-activation. To accomplish the linear precursor of pipecolidepsin A, the last two residues were introduced as one unit ( Supplementary Fig. S4 ) using PyBOP/HOAt/DIEA [29] in DMF to minimize C -terminus epimerization and prevent guanidinylation when HATU is used at longer times (3.5 h were required). After simultaneous Allyl and Alloc elimination with Pd(PPh 3 ) 4 in the presence of the scavenger PhSiH 3 , macrolactamization took place smoothly with PyBOP/HOAt/DIEA on solid phase for 3 h. Final cleavage and global deprotection of the peptide resin were carried out with trifluoroacetic acid (TFA)−H 2 O−TIS (95:2.5:2.5) in 1.5 h. The crude peptide was purified by semi-preparative reversed-phase high-performance liquid chromatography (HPLC) to furnish pipecolidepsin A with a purity over 95% and an overall yield of 3.3%. The synthetic peptide co-eluted with the natural one ( Supplementary Fig. S5 ) and NMR comparison revealed the spectroscopic equivalence of the two compounds ( Supplementary Tables S6 and S7 ). 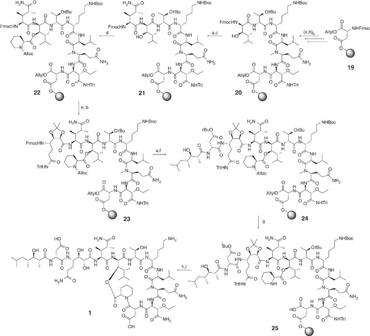Figure 4: Pipecolidepsin A solid-phase synthesis. (a) Piperidine−DMF (1:4) (2 × 1, 2 × 5, 1 × 10 min); (b) Fmoc-aa-OH, HATU, HOAt, DIEA and DMF, 1 h; (c) Fmoc-diMeGln-OH, DIPCDI, HOBt, DMF, 1 h; (d) Alloc-pipecolic-OH26, DIPCDI, DMAP, DCM−DMF, 45 °C, 2.3 h; (e) Piperidine−DMF (1:4) (2 × 2 min); (f) HTMHA-D-Asp(tBu)-OH37, PyBOP, HOAt, DIEA, DMF, 3.5 h; (g) Pd(PPh3)4, PhSiH3, dry DCM (3 × 15 min); (h) PyBOP, HOAt, DIEA, DMF, 3 h; and (i) TFA−H2O−TIS (95:2.5:2.5), 1.5 h. Figure 4: Pipecolidepsin A solid-phase synthesis. ( a ) Piperidine−DMF (1:4) (2 × 1, 2 × 5, 1 × 10 min); ( b ) Fmoc-aa-OH, HATU, HOAt, DIEA and DMF, 1 h; ( c ) Fmoc-diMeGln-OH, DIPCDI, HOBt, DMF, 1 h; ( d ) Alloc-pipecolic-OH 26 , DIPCDI, DMAP, DCM−DMF, 45 °C, 2.3 h; ( e ) Piperidine−DMF (1:4) (2 × 2 min); ( f ) HTMHA- D -Asp( t Bu)-OH 37 , PyBOP, HOAt, DIEA, DMF, 3.5 h; ( g ) Pd(PPh 3 ) 4 , PhSiH 3 , dry DCM (3 × 15 min); ( h ) PyBOP, HOAt, DIEA, DMF, 3 h; and ( i ) TFA−H 2 O−TIS (95:2.5:2.5), 1.5 h. Full size image Biological evaluation and insights into the mode of action Synthetic pipecolidepsin A was evaluated in vitro against three human tumour cell lines: lung (A549), colon (HT29) and breast (MDA-MB-231). A colorimetric assay, using sulforhodamide B reaction, was adapted to provide a quantitative measurement of cell growth and viability. Analysis of the dose–response data obtained from the assays afforded the GI 50 values (concentration of compound inducing a 50% reduction of cell growth [30] ) detailed in Table 1 . These values showed that both natural and synthetic peptides displayed comparable antiproliferative activity. The scaling up of pipecolidepsin A synthesis provided the DADHOHA deletion by-product ( Supplementary Fig. S6 ) in a sufficient amount to allow its HPLC-photodiode array (PDA) and HPLC-mass spectrometry (MS) characterization and biological evaluation. A longer Fmoc-deprotection treatment for the diMe-Gln moiety (2 × 2 min instead of 1 × 3 min) efficiently decreased the occurrence of this deletion. The biological results obtained for this side product are also included in Table 1 . Table 1 Biological evaluation. Full size table Further experiments were undertaken with natural pipecolidepsin A. Using a panel of 24 cell lines representative of 11 tissues, the peptide showed GI 50 values between 0.1 and 1 μM ( Supplementary Table S8 ) in a 72-h experiment. Interestingly, when A549 tumour cells were treated with the compound at a concentration of 3 μM, for as little as 30 min, >50% of cell death was observed in dose–response curves ( Fig. 5a ). At the morphological level, pipecolidepsin A had rapid and drastic effects on tumour cells. A few minutes after treatment of A549 lung adenocarcinoma cells with effective concentrations of the compound, the cells experienced rapid plasma membrane permeabilization, detected by internalization of propidium iodide (PI), as well as morphological changes characterized by severe cell swelling, the appearance of membrane blebs and the formation of giant vesicles ( Fig. 5b ). 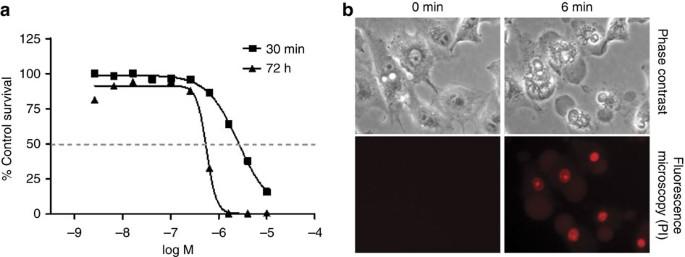Figure 5: Pipecolidepsin A induced permeabilization and cytotoxicity. (a) Representative cytotoxicity dose–response curves of pipecolidepsin A in A549 human lung adenocarcinoma cells after short (30 min, black squares) and long (72 h, black triangles) treatments. Cell viability was analysed and expressed as percentage of control cell survival. The IC50calculated were 2.62E−06 and 0.53E−06 M for short and long treatments, respectively. (b) A549 cells were treated or not with 1 μM pipecolidepsin A for 6 min in the presence of PI and analysed by phase contrast and fluorescence microscopy. Before addition of the compound, the cells were not permeable to PI; upon pipecolidepsin A addition, cells rapidly lost membrane integrity and became permeable to the dye, as evidenced by the strong nuclear staining (red fluorescence). Figure 5: Pipecolidepsin A induced permeabilization and cytotoxicity. ( a ) Representative cytotoxicity dose–response curves of pipecolidepsin A in A549 human lung adenocarcinoma cells after short (30 min, black squares) and long (72 h, black triangles) treatments. Cell viability was analysed and expressed as percentage of control cell survival. The IC 50 calculated were 2.62E−06 and 0.53E−06 M for short and long treatments, respectively. ( b ) A549 cells were treated or not with 1 μM pipecolidepsin A for 6 min in the presence of PI and analysed by phase contrast and fluorescence microscopy. Before addition of the compound, the cells were not permeable to PI; upon pipecolidepsin A addition, cells rapidly lost membrane integrity and became permeable to the dye, as evidenced by the strong nuclear staining (red fluorescence). Full size image The structure of pipecolidepsin A was determined by a combination of mono- and bi-dimensional NMR experiments and LC-MS analysis of the amino acid fragments obtained by hydrolysis and derivatization. However, some uncertainty concerning the stereochemical configuration of the two most demanding units, AHDMHA and DADHOHA, remained. Thus, more versatile synthetic strategies to access all possible diastereomers of these moieties were designed. For the DADHOHA moiety, NMR data from the natural pipecolidepsin A established S as the absolute configuration of C4 and suggested that C2 and C3 have the same configuration. Nevertheless, no spectroscopic data provided evidence of the relative configuration between the adjacent hydroxyl and amino groups at C3 and C4. Marfey’s analysis confirmed S as the absolute configuration for C4 but did not shed light on the stereochemistry of C2 and C3. Thus, a non-diastereoselective synthesis of DADHOHA starting from the commercially available Z- L -Gln(Trt)-OH was undertaken ( Fig. 2 ). The two hydroxyl substituents with the same configuration made it necessary to perform a cis -dihydroxylation, which was carried out non-stereoselectively using NMO and catalytic OsO 4 . Following this synthetic strategy, diastereomers (2 R ,3 R ,4 S ) and (2 S ,3 S ,4 S ) were obtained with 15% and 19% yields, respectively, after eight synthetic steps. A literature description of related residues found in other head-to-side-chain cyclodepsipeptides led us to consider the (2 R ,3 R ,4 S ) diastereomer as the preferred one. Also, stereochemical information regarding the unprecedented residue AHDMHA remained unclear. As the junction between the C -terminus and the peptide side chain via the β-hydroxy group, this amino acid is crucial in pipecolidepsins and homophymines. In pipecolidepsin A, its absolute configuration was assumed to be like that described for homophymine A, (2 R ,3 R ,4 R ), a hypothesis also supported by the preponderant D -allo isomerism of the residues ( D -allo -Thr, D -allo -β-hydroxy-Leu) found at the branching position of related natural head-to-side-chain cyclodepsipeptides. Despite this, an efficient stereoselective synthesis that allowed access to the four possible diastereomers (configuration at C2 remained fixed) was developed ( Fig. 3 , the complete synthesis of the four diastereomers will be published soon). After preparing all the building blocks required, we designed a synthetic process taking into account the possible side reactions and synthetic challenges that could be encountered, which are highlighted in Fig. 6 . 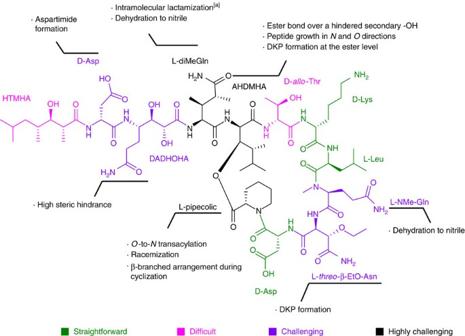Figure 6: Side reactions and synthetic challenges of pipecolidepsin A. [a]The formation of the dimethyl lactam also occurs in nature, as analogs of these peptides terminated with the dimethylpyroglutamic acid have been isolated38. Figure 6: Side reactions and synthetic challenges of pipecolidepsin A. [a] The formation of the dimethyl lactam also occurs in nature, as analogs of these peptides terminated with the dimethylpyroglutamic acid have been isolated [38] . Full size image First of all and considering the complexity of pipecolidepsin A structure, the strategy proposed was based on the safer Fmoc chemistry rather than the more harsh Boc chemistry. As the starting point for peptide elongation, the D -Asp residue in the cycle was chosen on the basis of the following advantages: (i) possibility of carrying out macrolactamization in both solid phase and solution; (ii) ester bond construction at a later stage of the peptide synthesis; (iii) attenuation of DKP formation involving both N -alkyl amino acids and esters within the chain; and (iv) minimal β-branched peptide elongation. Moreover, taking into account the steric hindrance of the amino acids of the sequence, the most potent HATU/HOAt/DIEA [31] system was adopted as the coupling system for the amide formation. 2-Chlorotrityl resin [32] , [33] was used as the solid support in the first attempts; however, this support was finally replaced by the more resistant Wang-like resin [3-(4-hydroxymethylphenoxy)propionylaminopolystyrene] [34] , as total cleavage of the peptide during ester formation was detected when scaling up the synthesis using 2-chlorotrityl resin. This resin is cleaved under very mild acid conditions, whereas Wang resin requires stronger acid conditions. The use of Wang resin precludes the need for the macrolactamization step in solution because the cleavage of the peptide—anchored through the α-carboxyl group of the D -Asp residue in the cycle—from the resin concomitantly removes all protecting groups. Given that the ester bond formation is the bottleneck of pipecolidepsin A synthesis, its construction at different peptide assembly stages was evaluated: after incorporation of Fmoc- D -allo -AHDMHA-OH, after Fmoc-diMeGln-OH or after Fmoc-DADHOHA(acetonide,Trt)-OH. The synthesis of the linear precursor until the Fmoc- D -allo -AHDMHA-OH moiety proceeded smoothly. No DKP formation was detected, and the percentage of the dehydrated by-product at the N Me-Gln residue was minor (<5%), despite using the strong HATU/HOAt/DIEA coupling system. Ester bond formation at this stage (intermediate 20 , Fig. 4 ) was quantitative when using DIPCDI and DMAP at 25 °C and long times (2 × 3 h, 1 × 12 h) (structure not shown in Fig. 4 ). Despite the bulky D -allo -AHDMHA side chain, a rapid O -to- N transacylation occurred (up to 50%) during the removal of its Fmoc group. This O -to- N transacylation occurs even when the deprotection is performed by means of a single 3-min treatment [35] . Performing the macrolactamization step after ester bond formation over intermediate 20 and before exocyclic arm elongation did not prevent the occurrence of this severe side reaction. The rigidity of the cycle was thought to jeopardize the O -to- N transacylation in a conformationally restricted mobility protection scheme [36] . However, the mass corresponding to a cyclized and transacylated product was detected in the complex peptide crude. Thus, this strategy was discarded, and elongation of the peptide chain until Fmoc-diMeGln-OH and before ester bond formation was evaluated. Fine tuning of the Fmoc-diMeGln-OH coupling conditions was needed to minimize the grave dehydration side reaction of the side-chain amide into a nitrile group, while keeping an excellent coupling yield. Thus, the neutral and mild DIPCDI/HOBt (11% of dehydrated by-product) proved to be the most suitable condition over a number involving the presence of base (HATU/HOAt/DIEA) or more acidic additives (DIPCDI/HOAt, DIPCDI/Oxyma). The reaction time and the equivalents were also crucial. One hour of reaction using 4.5 eq. provided quantitative couplings with minimized dehydration. A longer reaction treatment would represent a significant increase in the extent of dehydration, and fewer equivalents would require re-coupling. Finally, and as expected, no acylation of the unprotected D -allo -AHDMHA hydroxyl group was detected under any condition. Next, the esterification step over intermediate 21 ( Fig. 4 ) was evaluated to find suitable conditions that allowed good yields and prevented earlier removal of the Fmoc group of the diMeGln residue and, consequently, formation of the dimethylpyroglutamic derivative (see below).Thus, the final choice was a delicate balance between overcoming the added steric hindrance caused by the presence of the Fmoc-diMeGln residue, the loss of Fmoc when forcing conditions, and posterior fine tuning of the conditions to remove the Fmoc from diMeGln and to incorporate the subsequent Fmoc-DADHOHA(acetonide,Trt)-OH. A number of active species were generated, but only two conditions, aa−DIPCDI−DMAP (10:10:0.5) and the symmetrical anhydride ( Supplementary Table S9 ), furnished the desired intermediate 22 . Nevertheless, to achieve quantitative conversions with reasonable purity, it was crucial to apply temperature, aa–DIPCDI–DMAP being the most reactive, and therefore providing the most satisfactory results. Alloc-pipecolic-OH 26 (15 eq. ), DIPCDI (15 eq. ), DMAP (0.5 eq.) and DCM−DMF (9:1), 45 °C, 2.3 h, were the final optimized conditions. Ester bond formation after incorporation of the residue Fmoc-DADHOHA(acetonide,Trt)-OH could not be achieved under any conditions, including harsh treatments at high temperatures or strong heating using MW. Thus, this third strategy was ruled out. Elimination of the Fmoc group of the diMeGln residue and incorporation of the Fmoc-DADHOHA(acetonide,Trt)-OH was also a tricky transformation, as once the Fmoc group was removed, an intramolecular cyclization took place, rendering the corresponding lactam (pyrodiMeGlu) and truncating the peptide chain elongation. This by-product was detected only when analysing unprotected compound 23 ( Fig. 4 ). Thus, optimized conditions with minimized by-products and maximum conversions to obtain intermediate 23 involved temperatures around 45 °C for the ester formation (entry 6, Supplementary Table S9 ), rapid Fmoc elimination (2 × 2 min) and a 1-min pre-activation of the incoming Fmoc-DADHOHA(acetonide,Trt)-OH with HATU/HOAt/DIEA ( Fig. 4 ). The absence of pre-activation led to a higher formation of the by-product terminated with the pyrodiMeGlu. Stepwise incorporation of Fmoc- D -Asp( t Bu)-OH and HTMHA resulted in more complex crude profiles, probably as a result of aspartimide formation. To avoid this side reaction, these last two moieties were introduced as a pseudodipeptide, providing cleaner crudes. The Allyl and the Alloc groups were then removed, and the macrolactamization step was carried out on solid phase using PyBOP/HOAt/DIEA in DMF for 3 h. Exhaustive exploration of HPLC-PDA conditions led to a planar gradient, which enabled purification of the final crude, providing synthetic pipecolidepsin A with a purity >95%. Chemical, spectral and biological equivalence of synthetic and natural pipecolidepsin A was proved by HPLC-PDA co-elution ( Supplementary Fig. S5 ), NMR comparison ( Supplementary Tables S6 and S7 ) and biological evaluation of the two compounds ( Table 1 ). The proved equivalence served to validate the synthetic strategy and to demonstrate that (2 R ,3 R ,4 R )-AHDMHA and (2 R ,3 R ,4 S )-DADHOHA were, as predicted, the diastereomers sharing the same stereochemistry with the corresponding moieties in the natural peptide. Finally, the membrane permeabilization assays and the morphological changes observed by phase contrast microscopy indicated that pipecolidepsin A induced a lytic process that leads to rapid necrotic cell death. Given that the cellular effects observed with pipecolidepsin A are quite similar to those detected with the structurally related compound Irvalec [37] , it is likely that these compounds share a common mechanism of action, directly interacting with the plasma membrane of tumour cells. Interestingly, the cyclodepsipeptide lacking the diol (DADHOHA) moiety did not show any cytotoxicity, thereby highlighting the relevance of the linear peptidic arm and pointing out the importance of the distinctive head-to-side-chain scaffold in the biological activity of these natural products. In summary, here we report on the first total synthesis of a D -allo -AHDMHA containing head-to-side-chain cyclodepsipeptide on solid phase, thereby providing confirmation of all stereocenter configurations. After successfully performing the synthesis of the suitably protected key building blocks DADHOHA and AHDMHA, the formation of the key ester bond over an extremely hindered secondary alcohol was also achieved with minimized by-products. The robust synthetic route overcame all the side reactions associated with these structurally complex peptides and led to the desired natural product. This strategy may be of general application to other related cyclodepsipeptides that have pharmacological properties of interest, like those described herein. Reagents and solvents Protected amino acid derivatives were obtained from Bachem and Iris-Biotech. Coupling reagents, linkers and resins were purchased from MedalChemy, Aldrich, Luxembourg Industries and NovaBiochem. Solvents and piperidine were obtained from SDS. Reagents of common use were obtained from Aldrich and Panreac. All commercial reagents and solvents were used as received. HPLC-PDA and HPLC-MS Analytical HPLC-PDA was performed on a Waters instrument comprising a separation module (Waters 2695), an automatic injector, a photodiode array detector (Waters 996 or Waters 2998) and a system controller (Millenium [31] login). The columns used were Xbridge C18 reversed-phase analytical column (2.5 μm × 4.6 mm × 75 mm) and Xbridge BEH130 C18 reversed-phase analytical column (3.5 μm × 4.6 mm × 100 mm). Ultraviolet detection was at 220 and 254 nm, and linear gradients of acetonitrile (ACN) (+0.036% TFA) into H 2 O (+0.045% TFA) were run at a 1 ml min −1 flow rate over 8 min. Semi-analytical HPLC was carried out on the same Waters instrument but using a Xbridge Prep BEH130 C18 reversed-phase column (5 μm × 10 mm × 100 mm) and linear gradients with a flow rate of 3 ml min −1 over 20 min. HPLC-MS analysis was performed on a Waters instrument comprising a separation module (Waters 2695), an automatic injector, a photodiode array detector (Waters 2998), a Waters Micromass ZQ spectrometer and a system controller (Masslynx v4.1). The column used was a Sunfire C18 reversed-phase analytical column (3.5 × 2.1 × 100 mm 3 ). Ultraviolet detection was at 220 and 254 nm, and linear gradients of ACN (+0.07% Formic acid) into H 2 O (+0.1% Formic acid) were run at a 0.3 ml min −1 flow rate over 8 min. NMR 1 H and 13 C NMR spectra were recorded on a Varian MERCURY 400 (400 MHz for 1 H NMR, 100 MHz for 13 C NMR) spectrometer, 500 MHz NMR Varian Unit Inova 500 spectrometer and on a Bruker 600 Avance III Ultrashielded spectrometer, provided with a cryoprobe TCI (600 MHz for 1 H NMR, 150 MHz for 13 C NMR). Chemical shifts ( δ ) are expressed in parts per million downfield from tetramethylsilane chloride. Coupling constants are expressed in Hertz. Cell lines and viability assays A panel of cell lines was used representing the following cancerous tissue types: prostate (PC-3 and 22Rv1), pancreas (PANC-1 and MiaPaca-2), ovary (IGROV-1 and A2780), sarcoma (SAOS2), lung (NCI-H460, NCI-H23 and A549), liver (SK-HEP-1 and HepG2), leukaemia (MOLT-4 and K-562), renal (RXF 393 and Caki-1), gastric (HGC-27 and HS 746T), colon adenocarcinoma (LoVo, HT29 and HCT-116) and breast (MDA-MB-231, MCF-7 and BT-474). Cells were seeded in 96-well microtiter plates and allowed to stand for 24 h at 37 °C and 5% CO 2 in drug-free medium before treatment with vehicle alone or pipecolidepsin A at the concentrations and times indicated in the text. For cell survival quantification, MTT was added to the cell cultures for 8 h. Then, the culture medium was carefully removed, and the coloured formazan crystals were dissolved in DMSO. The absorbance of the samples was measured at 540 nm using a microplate spectrophotometer. Results are expressed as percentage of control cell survival and represent the mean of at least three independent experiments. Membrane permeabilization assays For time-course experiments, cells were seeded at high density in 96-well clear-bottom black plates and cultured as described above. When confluence was reached, fresh culture medium (supplemented with 25 mM HEPES pH 7.4 and 50 mg ml −1 PI) containing or not a range of pipecolidepsin A concentrations was added. The uptake of PI was monitored by fluorescence microscopy. Synthesis of building blocks Solution reactions were performed in round-bottomed flasks. Organic layers were dried over anhydrous Na 2 SO 4 or MgSO 4 , and the solvent removed under reduced pressure at temperatures below 40 °C. All reactions were monitored by TLC on MERCK TLC plates silica gel 60F 254 under ultraviolet light (254 nm), and/or stained with ethanolic phosphomolybdic acid (12 g in 100 ml) or ninhydrin solution (1.5 g ninhydrin, 3 ml AcOH, 100 ml EtOH). Flash column chromatography was carried out using SDS Silica gel 60A (35–70 μm). Synthesis of (2 R ,3 R ,4 S )-Fmoc-DADHOHA(acetonide,Trt)-OH Commercially available Z- L -Gln(Trt)-OH was converted into the aldehyde 4 using the Weinreb amide method ( Supplementary Methods ). Then, a solution of 0.5 M of KHMDS in dry toluene (2.6 eq.) was added dropwise to a solution of 18-Crown-6 (4.4 eq.) and methyl P , P -bis(2,2,2-trifluoroethyl)phosphonoacetate (2.6 eq.) in dry tetrahydrofuran (THF) cooled to −78 °C and under Ar. After 30 min of stirring, a solution of aldehyde 4 (1 eq.) in dry THF was cannulated into the reaction mixture and allowed to react at −78 °C for 3 h. The alkene 5 was obtained with 67% yield. 4-Methylmorpholine N -oxide (NMO) (3 eq.) and OsO 4 (catalytic) were added to a solution of alkene 5 (1 eq.) in THF−H 2 O, and the resulting reaction mixture was stirred for 10 days at room temperature. The reaction was quenched with a 40% aqueous NaHSO 3 solution for 30 min. (2 R ,3 R ,4 S ) Diol 6 and (2 S ,3 S ,4 S ) diol 6b were obtained with 38% and 39% yield, respectively. The diols were protected as pentacyclic acetals, the methyl esters hydrolysed in basic media, the Z groups eliminated by hydrogenolysis and the resulting free amines suitably protected with a Fmoc group. Final (2 R ,3 R ,4 S )-Fmoc-DADHOHA(acetonide,Trt)-OH 10 was obtained with 15% yield after eight steps. 1 H NMR (400 MHz, CD 3 OD) δ 1.35 (s, CH 3, dioxolane, 3H), 1.57 (s, CH 3 , dioxolane, 3H), 1.76 (m, CH 2 2’ , 1H), 1.88 (m, CH 2 2′ , 1H), 2.29 (m, CH 2 3′ , 2H), 4.01 (m, CH 1′ , 1H), 4.24 (dd, J =6.9, 6.9 Hz, CH, Fmoc, 1H), 4.33 (m, CH 2 , Fmoc, 2H), 4.38 (m, CH 5 , 1H), 4.62 (d, J =7.6 Hz, CH 4 , 1H), 7.16–7.31 (m, Fmoc, Trt, 17H), 7.37 (dt, J =7.4, 7.4, 3.3 Hz, CH, Ar, Fmoc, 2H), 7.64 (d, J =7.3 Hz, CH, Ar, Fmoc, 1H), 7.69 (d, J =7.4 Hz, CH, Ar, Fmoc, 1H), 7.78 (d, J =7.5 Hz, CH, Ar, Fmoc, 2H); 13 C NMR (400 MHz, CD 3 OD) δ 24.86 (CH 3 , dioxolane), 26.82 (CH 3 , dioxolane), 30.99 (CH 2 2′ ), 34.67 (CH 2 3′ ), 49.33 (CH, Fmoc), 51.53 (CH 1′ ), 67.95 (CH 2 , Fmoc), 71.61 (Cq, Trt), 77.00 (CH 4 ), 80.43 (CH 5 ), 110.73 (Cq, dioxolane), 120.92 (CH, Ar, Fmoc), 126.37 (CH, Ar, Fmoc), 126.59 (CH, Ar, Fmoc), 127.74 (CH, Ar, Trt), 128.19 (CH, Ar, Fmoc), 128.70 (CH, Ar, Trt), 128.75 (CH, Ar, Fmoc), 128.82 (CH, Ar, Fmoc), 130.08 (CH, Ar, Trt), 142.55 (Cq, Fmoc), 142.70 (Cq, Fmoc), 145.11 (Cq, Fmoc), 145.83 (Cq, Fmoc), 146.09 (Cq, Ar, Trt), 158.71 (OCONH), 174.92 (CO); and HRMS (NanoESI) m/z calculated for C 44 H 43 N 2 O 7 (M+H) + 711.3065, found 711.3077 ( Supplementary Figs S7–S12 for diastereomer 10b ). Synthesis of (2 R ,3 R ,4 R )-Fmoc-AHDMHA-OH A 1.7 M solution of tert -butyl lithium in hexane (4 eq.) was added dropwise over 20 min to a pre-cooled solution of 2-bromo-3-methyl-but-2-ene (4 eq.) in dry Et 2 O at −78 °C ( Supplementary Methods ). The resulting mixture was stirred for 3 h. Then a solution of Garner’s aldehyde 12 (1 eq.) in dry Et 2 O was added over 1 h, and the mixture was warmed up to room temperature and stirred overnight. Saturated aqueous NH 4 Cl was used to quench the reaction. Olefin 13 was obtained with 36% yield. After its reduction, the resulting intermediate 14 (1 eq.) was dissolved with 2,6-di- tert -butyl pyridine (2.2 eq.) in dry DCM, and Tf 2 O was added at 0 °C. The resulting pulp was stirred for 10 min. Oxidation with Jones reagent at 0 °C in acetone provided the desired cyclic carbamate 16 . Acid hydrolysis of 16 and protection with the Fmoc group furnished the desired (2 R ,3 R ,4 R )-Fmoc-AHDMHA-OH 18 with 15% overall yield after six steps. α D 25 =−5.8 ( c =1.0, CHCl 3 ); mp 90–93 °C; 1 H NMR (acetone- d6 ) δ 7.86 (d, J =7.5 Hz, 2H), 7.73 (m, 2H), 7.42 (m, 2H), 7.33 (m, 2H), 6.54 (d, J =8.9 Hz, 1H), 4.49 (m, 1H), 4.36 (m, 2H), 4.25 (m, 1H), 3.71 (dd, J =9.7, 2.7 Hz, 1H), 2.25 (m, 1H), 1.85 (m, 1H), 0.92 (d, J =7.0 Hz, 3H), 0.89 (d, J =6.9 Hz, 3H) and 0.79 (d, J =6.9 Hz, 3H); 13 C NMR (acetone- d6 ) δ 172.8, 157.8, 146.0, 143.1, 129.5, 128.9, 127.1, 121.8, 77.3, 68.3, 58.9, 49.0, 42.3, 28.0, 22.9, 16.6 and 11.0; and HRMS (NanoESI) m/z calculated for C 23 H 28 NO 5 [M+H] + 398.1962, found 398.1974 ( Supplementary Figs S13–S15 ). Synthesis of Alloc-pipecolic-OH 26, HTMHA, HTMHA- D -Asp( t Bu)-OH and pipecolidepsin A Solid-phase syntheses were undertaken in polypropylene syringes fitted with two polyethylene filter discs ( Supplementary Methods ). All solvents and soluble reagents were removed by suction. Washings between deprotection, coupling and cyclization steps were carried out with DMF (3 × 1 min) and DCM (3 × 1 min) using 4 ml solvent for each wash. When not specified, all transformations and washes were performed at 25 °C. Aminomethyl resin (0.36 mmol g −1 ) was used. The linker 3-(4-hydroxymethylphenoxy)propionic acid was introduced using HBTU-HOBt-DIEA (3:3:9) in DMF for 1.5 h. General coupling conditions: aa−HATU−HOAt−DIEA (1:1:1:2) in DMF for 1 h with 1 min of pre-activation. General deprotection conditions: piperidine–DMF (1:4) (2 × 1 min, 2 × 5 min and 1 × 10 min). Coupling conditions for Fmoc-diMe-Gln-OH: aa–DIPCDI–HOBt (4.5:4.5:4.5) in DMF for 1 h without pre-activation. Deprotection conditions for Fmoc-diMe Gln-OH: piperidine–DMF (1:4) (2 × 2 min). Ester bond formation conditions: Alloc–pipecolic–OH–DIPCDI–DMAP (15:15:0.5), dry DCM–dry DMF (9:1), 45 °C, 2.3 h. The reagents were mixed at 0 °C and filtered before being added to the resin. Coupling conditions for HTMHA- D -Asp( t Bu)-OH: pseudodipeptide-PyBOP-HOAt-DIEA (5:5:5:10) in DMF for 3.5 h without pre-activation. Allyl and Alloc deprotection conditions: Pd(PPh 3 ) 4 -PhSiH 3 (0.1:10) in dry DCM, under N 2 , 3 × 15 min. Cyclization conditions: PyBOP-HOAt-DIEA (4:4:8) in DMF for 3 h. Cleavage and final deprotection conditions: TFA–H 2 O–TIS (95:2.5:2.5) for 1.5 h. Purification conditions: XBridge Prep BEH130 C18 (5 μm × 10 mm × 100 mm) column and a linear gradient (5–35% over 5 min and 35–37% over 20 min) of ACN (0.036% TFA) into H 2 O (0.045%) with a flow rate of 3.0 ml min −1 ( t R =14.13 min) to give pipecolidepsin A in 3.3% yield. HRMS(NanoESI) analysis showed the following: m/z calculated for C 37 H 64 O 13 N 8 828.4587 [(M+2H)/2] 2+ , found 828.4583 ( Supplementary Fig. S16 ). The product co-eluted by HPLC-PDA with a natural sample of pipecolidepsin A ( Supplementary Fig. S5 ). Conditions: linear gradient (36–38%) of ACN (0.036% TFA) into H 2 O (0.045%) over 40 min, with a flow rate of 1.0 ml min −1 ( t R =19.53 min) in a Phenomenex Column C18 (5 μm × 4.6 mm × 250 mm). The 1 H NMR (600 MHz, CD 3 OH) spectrum of the synthetic peptide perfectly matched with the natural one ( Supplementary Figs S17–S26 and Supplementary Tables S6 and S7 ). For further experimental details, check intermediate characterization and NMR spectra in the Supplementary Methods . Accession codes: The X-ray crystallographic coordinates for structures reported in this article have been deposited at the Cambridge Crystallographic Data Centre (CCDC), under deposition number CCDC 933496. These data can be obtained free of charge from The Cambridge Crystallographic Data Centre via www.ccdc.cam.ac.uk/data_request/cif . How to cite this article: Pelay-Gimeno, M. et al. The first total synthesis of the cyclodepsipeptide pipecolidepsin A. Nat. Commun. 4:2352 doi: 10.1038/ncomms3352 (2013).